Accessing 4f-states in single-molecule spintronics Magnetic molecules are potential functional units for molecular and supramolecular spintronic devices. However, their magnetic and electronic properties depend critically on their interaction with metallic electrodes. Charge transfer and hybridization modify the electronic structure and thereby influence or even quench the molecular magnetic moment. Yet, detection and manipulation of the molecular spin state by means of charge transport, that is, spintronic functionality, mandates a certain level of hybridization of the magnetic orbitals with electrode states. Here we show how a judicious choice of the molecular spin centres determines these critical molecule–electrode contact characteristics. In contrast to late lanthanide analogues, the 4 f -orbitals of single bis(phthalocyaninato)-neodymium(III) molecules adsorbed on Cu(100) can be directly accessed by scanning tunnelling microscopy. Hence, they contribute to charge transport, whereas their magnetic moment is sustained as evident from comparing spectroscopic data with ab initio calculations. Our results showcase how tailoring molecular orbitals can yield all-electrically controlled spintronic device concepts. Molecular spintronics combine the auspicious characteristics of molecular electronics [1] , [2] and spintronics [3] to exploit the rich diversity and functionality of molecules, and the spin degree of freedom for novel nanoelectronic device concepts [4] , [5] , [6] . An effective approach to molecular spintronics is the investigation of discrete magnetic molecules in contact with metallic leads [7] . In this context, lanthanide (Ln)-based bis(phthalocyaninato)-Ln(III) complexes (LnPc 2 ) represent a promising class of stable and redox-active molecules. For instance, the magnetic properties of TbPc 2 were investigated on non-magnetic [8] , [9] , [10] as well as on magnetic [11] , [12] surfaces. However, the 4 f -electrons in the late Ln, such as Tb or Dy, lie deep in energy and are spatially localized around the nucleus and, thus, do not contribute to charge transport. Access to the 4 f -states in charge-transport experiments thus require them to be closer to the Fermi level and less localized so as to hybridize with the molecular orbitals of the ligands, all of which are met only for the early Ln. Of similar importance is the modification of the electronic structure and notably the magnetism of a magnetic molecule caused by the adsorption on an electrode [13] , [14] , [15] , [16] , [17] , [18] . Here we address these key issues and present the results of a combined experimental and theoretical study of bis(phthalocyaninato)-neodymium(III) (NdPc 2 ) adsorbed on the Cu(100) surface, a successful model system for a molecule–electrode contact with accessible spin-polarized 4 f -states. In contrast to, for example, a Tb 3+ ion with an electronic configuration [Xe]4 f 8 6 s 0 , the Nd 3+ ion ([Xe]4 f 3 6 s 0 ) has a larger ionic radius (112 versus 104 pm) with more delocalized 4 f -electrons and, thus, stronger hybridization with the phthalocyanine ligands. Thereby, the 4 f -orbitals become accessible to transport experiments, while largely maintaining the relative energetic positions of spin-up/-down states and consequentially the magnetic moment. Adsorption configuration of NdPc 2 on Cu(100) The approximately D 4d -symmetric double-decker structure of the NdPc 2 molecule is shown in Fig. 1a . One of the two Pc ligands chemisorbs the molecule in a flat geometry on the Cu(100) surface, whereas the second Pc, exposed to vacuum, retains its molecular-type electronic features. 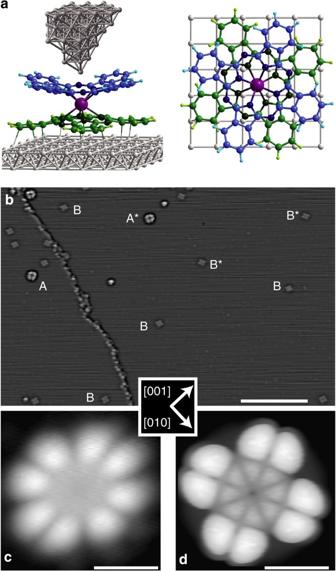Figure 1: Geometry and adsorption configuration of NdPc2on Cu(100). (a) Calculated adsorption geometry of the double-decker structure (light grey, Cu; dark grey, W; magenta, Nd; blue and green, Pc ligands; with N dark, C medium, H light colour). (b) STM overview showing isolated intact double-decker NdPc2(A/A*) and decomposed single-decker Pc or NdPc (B/B*) molecules. Two adsorption sites A/A* and B/B* are identified for both species, respectively. Scale bar, 20 nm. (c) STM topography of an NdPc2molecule and (d) the corresponding calculated STM image. Scale bars incandd, 1 nm. The used tunnelling parameters areItunnel=2 nA,Vbias=−1 V inbandItunnel=2 nA,Vbias=−0.8 V inc. The topography indis calculated for the energyE–EF=−0.8 eV. Figure 1b shows a scanning tunnelling microscopy (STM) overview image of NdPc 2 molecules adsorbed on the Cu(100) surface. The in-house synthesized crystalline evaporant exclusively consisted of NdPc 2 as confirmed by ultraviolet–visible absorption spectroscopy and mass spectrometry. Double-decker molecules and single-decker Pc molecules with or without the central Nd ion were identified by shape and height. Note that the low stability of NdPc 2 compared with its late Ln analogues originates from its larger Ln ionic radius [19] . Both double-decker (label A in Fig. 1b ) and single-decker (label B) species adsorb in two degenerate orientations (marked with or without a star) on the Cu(100) surface. For single-decker and double-decker species, the two orientations differ by an in-plane angle of 52°, in line with results for CuPc (ref. 20 ). Our ab initio calculations show that in the energetically most favourable adsorption geometry, the central Nd ion lies above the Cu(100) hollow site ( Fig. 1a ). In our STM studies, the two adsorption configurations A and A* are observed as equivalent and exhibit identical electronic features. In the following, we focus on NdPc 2 molecules in the adsorption configuration A shown in Fig. 1c . Figure 1: Geometry and adsorption configuration of NdPc 2 on Cu(100). ( a ) Calculated adsorption geometry of the double-decker structure (light grey, Cu; dark grey, W; magenta, Nd; blue and green, Pc ligands; with N dark, C medium, H light colour). ( b ) STM overview showing isolated intact double-decker NdPc 2 (A/A*) and decomposed single-decker Pc or NdPc (B/B*) molecules. Two adsorption sites A/A* and B/B* are identified for both species, respectively. Scale bar, 20 nm. ( c ) STM topography of an NdPc 2 molecule and ( d ) the corresponding calculated STM image. Scale bars in c and d , 1 nm. The used tunnelling parameters are I tunnel =2 nA, V bias =−1 V in b and I tunnel =2 nA, V bias =−0.8 V in c . The topography in d is calculated for the energy E – E F =−0.8 eV. Full size image The NdPc 2 molecule appears in STM topography images as an eight-lobe shape with a fourfold symmetry as previously observed for late lanthanide double-decker species [8] , [9] . The STM image mainly reflects the charge distribution of the upper Pc ring. Each two-lobe feature is attributed to one benzene subgroup [8] and is also observed in STM images of non-coordinated Pc molecules on insulating surfaces [21] . This similarity indicates that for NdPc 2 /Cu(100), the chemisorption does not significantly alter the molecular electronic features of the upper Pc ligand. The calculated STM image depicted in Fig. 1d reproduces the experimental topography in detail. For other bias voltages than in Fig. 1c,d , the STM topography images slightly change, but all characteristics are reproduced by the corresponding theoretical STM images (see Fig. 4a–h ). 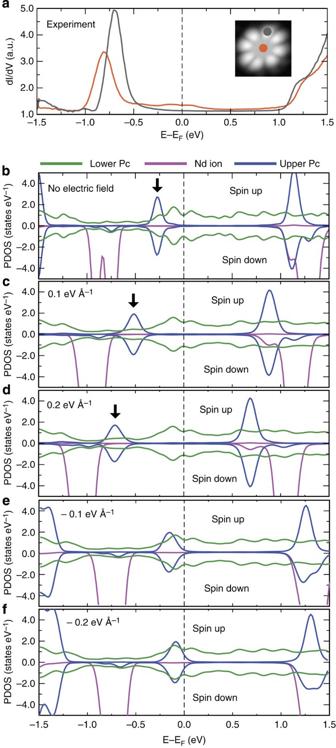Figure 2: Experimental dI/dVspectra and calculated PDOS. (a) Experimental dI/dVspectra measured at ligand (grey) and centre (orange) sites of the molecule. (b–f) Decomposition of the total spin-dependent PDOS into contributions from the lower Pc ring (green), the Nd ion (magenta; only 4f-states contribute in the displayed energy range) and the upper Pc ring (blue) calculated for different applied electric fields. Black arrows mark the occupied peak of the upper Pc ring that strongly shifts under the influence of the electric field. Ina, the tip is stabilized atItunnel=1 nA,Vbias=−1 V. Figure 2: Experimental d I /d V spectra and calculated PDOS. ( a ) Experimental d I /d V spectra measured at ligand (grey) and centre (orange) sites of the molecule. ( b – f ) Decomposition of the total spin-dependent PDOS into contributions from the lower Pc ring (green), the Nd ion (magenta; only 4 f -states contribute in the displayed energy range) and the upper Pc ring (blue) calculated for different applied electric fields. Black arrows mark the occupied peak of the upper Pc ring that strongly shifts under the influence of the electric field. 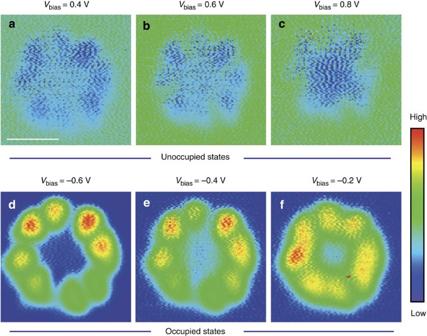Figure 3: Experimental dI/dVmaps confirm the shifting of the ligand states. The dI/dVmaps in the bias range from −0.6 to 0.8 V reveal a contrast inversion between unoccupied (a–c) and occupied (d–f) states. Scale bar ina, 1 nm. Ina,b,dande,Itunnel=1 nA, and incandf,Itunnel=0.5 nA. In a , the tip is stabilized at I tunnel =1 nA, V bias =−1 V. Full size image Figure 3: Experimental d I /d V maps confirm the shifting of the ligand states. The d I /d V maps in the bias range from −0.6 to 0.8 V reveal a contrast inversion between unoccupied ( a – c ) and occupied ( d – f ) states. Scale bar in a , 1 nm. In a , b , d and e , I tunnel =1 nA, and in c and f , I tunnel =0.5 nA. 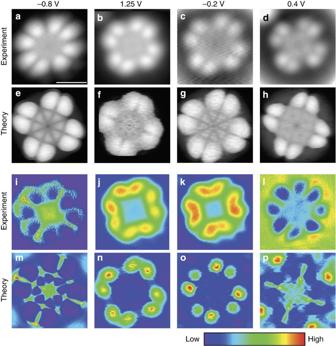Figure 4: Experimental and calculated topography images and dI/dVmaps. (a–d) Experimental and (e–h) theoretical topography images, (i–l) experimental and (m–p) theoretical dI/dVmaps for variousVbiasas indicated. Scale bar ina, 1 nm. Ina–dandi–l,Itunnel=1 nA. Full size image Figure 4: Experimental and calculated topography images and d I /d V maps. ( a – d ) Experimental and ( e – h ) theoretical topography images, ( i – l ) experimental and ( m – p ) theoretical d I /d V maps for var i ous V bias as indicated. Scale bar in a , 1 nm. In a – d and i – l , I tunnel =1 nA. Full size image Density of states of NdPc 2 on Cu(100) The hybrid NdPc 2 /Cu(100) electronic states are explored by performing d I /d V measurements at specific positions of the STM tip above the NdPc 2 molecule. d I /d V curves measured at the centre of the molecule and above the organic ligand are shown in Fig. 2a . Both spectra display two clear features near the Fermi energy E F . For the interpretation of the experimental d I /d V spectra and the calculated projected density of states (PDOS) in Fig. 2 , it is important to understand first the electronic structure of the free neutral NdPc 2 molecule. A total of three electrons, that is, two 6 s -electrons and one 4 f -electron, are formally transferred from the metal to the ligands, leading to an electrostatic interaction between Nd 3+ and the two negatively charged Pc rings. As a consequence, the Nd 3+ ion remains with three 4 f -electrons in one spin channel, whereas the two Pc ligands share one unpaired electron. Spin-polarized first-principles calculations for the adsorbed NdPc 2 on Cu(100) in Fig. 2b show for the lower Pc ring broad hybrid molecule-surface electronic states due to hybridization and charge transfer [17] , causing the magnetic moment on the ligands to vanish. The PDOS of the upper Pc ring (blue in Fig. 2b–d ), however, keeps sharp molecular-like features similar to those obtained for NdPc 2 in the gas phase [8] . This striking difference suggests that the two Pc rings are coupled via weak hybridization with the three 4 f -electrons through the Nd ion. This weak hybridization together with Hund’s rule constrain the Nd 3+ 4 f -electrons to be in the same spin channel, resulting in the spin magnetic moment. Therefore, the d I /d V peak measured on the centre site of the molecule (orange curve) for V bias =−0.8 V can be unequivocally assigned to an occupied electronic state with mainly 4 f -character in only the spin-down channel at the Nd site. For the same spectrum, the d I /d V shoulder measured for V bias =1.25 V perfectly matches the calculated PDOS for the unoccupied Nd spin-down 4 f -states at the same energy. As a result, in contrast to previously studied late LnPc 2 complexes [9] , [12] , the Nd 4 f -states can directly be accessed by STM. Similarly, we obtain good agreement between the d I /d V shoulder measured at the ligand site (grey curve) for V bias =+1.2 V and the unoccupied states with sharp PDOS features of the upper Pc ring. It is important to note that the Hubbard parameter for the 4 f -states ( U =2.2 eV) was chosen to reproduce the experimental d I /d V features for the occupied states in the centre of the molecule ( Fig. 2a ). This choice consistently leads to an exact match for the unoccupied states, too. Electric field-induced shifting of the ligand states Intriguingly, the agreement found for the positions of the 4 f -states does not seem to hold for the broad d I /d V peak measured at the ligand site for V bias ≈−0.7 V. The corresponding PDOS features, tentatively assigned to the upper Pc ring, are closer to the Fermi energy by ≈0.5 eV. This apparent mismatch manifests the largely conserved molecular-like features of the upper Pc ring and can be resolved by including an external electric field in our first-principles calculations, which represents the bias field in STM measurements. To assess the effect of such an electric bias field on the electronic structure of the NdPc 2 /Cu(100) system, a uniform field was taken into account ( Fig. 2b–f ), where positive (negative) electric fields are generated by negative (positive) bias voltages. Remarkably, a positive electric field effectively shifts the PDOS peak of the upper Pc ring located initially at ≈−0.2 eV to lower energies (black arrows in Fig. 2b–d ) until it gradually approaches the position of the occupied 4 f -derived peak. Under the influence of negative electric fields, the occupied PDOS peak of the upper Pc ring only shifts towards the Fermi level, but does not cross it. The unoccupied ligand peak shifts slightly from initially 1.1 to 1.3 eV, where is starts to overlap with the unoccupied 4 f -derived peak. Without electric field, the unoccupied ligand state is more strongly hybridized with the 4 f -state than the occupied counterpart. The stronger the hybridization, the less susceptible a state is to the electric field, resulting in a pinning at the energetic position of the hybridized state. Further support for the electric field-induced shifting of the ligand states stems from d I /d V maps measured at bias voltages between −0.6 and 0.8 eV shown in Fig. 3 . We do not detect any significant contribution of unoccupied states on the ligand sites ( Fig. 3a–c ) in accordance with the d I /d V versus V curve in Fig. 2a . In contrast, the d I /d V maps at negative bias ( Fig. 3d–f ) show spectral weight, which displays only minor changes in intensity and spatial distribution when varying the bias between −0.2 and −0.6 eV. This contribution can thus be related to the tail of the shifting peak in Fig. 2b–d . It is detectable as a spatial contrast in the d I /d V maps at bias voltages between 0 and −0.6 eV, but only shows up as a peak at −0.7 eV in the d I /d V versus V curve in Fig. 2a , when the corresponding ligand state is pinned by hybridization. Note, that this experimentally observed inversion of the d I /d V contrast between the occupied and unoccupied states in the V bias range from −0.6 to 0.8 V is reproduced in the first-principles calculations shown in Fig. 4 . Overall, the ability of the external electric field to shift the energetic position of the hybrid molecule-surface states with molecular character at the upper Pc ring is another specific aspect of the Nd 3+ coordination to this ring, which is primarily due to an electrostatic interaction modulated with a weak, yet significant hybridization between the 4 f and the ligand states. Notably, the inclusion of the electric field in our density functional theory simulations barely modified the energy position and the magnetic moment of the Nd 4 f -states, as they are spatially localized around the Nd core. This is also valid for the states of the lower Pc ring, which are strongly hybridized [17] with the Cu states. Comparison of measured and calculated d I /d V maps A direct contribution of the 4 f -states to the tunnelling current is further evidenced by the remarkable agreement between the experimental and simulated topography images, as well as the corresponding d I /d V maps shown Fig. 4 . Topography images correspond to isosurfaces of the local density of states integrated over all states between E F and eV bias , rendering simulated topography images rather robust. In contrast, the d I /d V maps represent only very few states in a narrow energy interval and, thus, are highly susceptible to small changes to relevant states. Note that the simulated d I /d V maps are evaluated at the isosurface of the corresponding topography image without further adjustments. Hence, our conclusions are based on the simultaneously achieved good agreement for both topographic images ( Fig. 4a–d versus Fig. 4e–h ) and d I /d V maps ( Fig. 4i–l versus Fig. 4m–p ). Slight changes of the apparent molecular shape in the experimental topographies for different energies ( Fig. 4a–d ) are well reproduced by the calculations ( Fig. 4e–h ). Although matching simulated and experimental d I /d V maps is more challenging, in particular the relative weights of the contributions from the ligand and centre sites are well reproduced ( Fig. 4i–p ). Overall, the extensive match between experiment and simulation confirms that the 4 f -states, which according to the calculated spin-resolved PDOS curves carry the spin magnetic moment, contribute to the transport through the molecule. In contrast to extensively studied analogous systems comprising late lanthanides, the spin-polarized 4 f -states are directly involved in electrical transport through NdPc 2 molecules in contact with a Cu(100) surface. The Nd 4 f -states are unambiguously identified based on their spectral position and spatial features by comparing scanning tunnelling spectroscopy and ab initio calculations. They are highly spin-polarized and, thus, carry the spin magnetic moment of the electrode-adsorbed molecule. Accessing these states by means of transport is expected to be a general feature of early Ln-based molecular magnets, where the 4 f -states are closer to the Fermi level and can be adjusted via coordination and surface interactions. This strategy opens up prospects for electrical manipulation and detection of the molecular spin state, providing the foundation for all-electrically controlled device concepts in molecular spintronics. Molecule synthesis NdPc 2 (refs 22 , 23 ) was prepared using the procedure reported by Weiss and coworkers [24] for the lutetium analogue and was used by Yamashita and coworkers [9] , [25] , [26] for the terbium, dysprosium and yttrium complexes, with modified purification steps. Phthalonitrile (8.0 g, 63 mmol), neodymium acetate hydrate (1.38 g, 4.0 mmol based on the composition Nd(CH 3 COO) 3 ·1.1H 2 O determined by thermogravimetric analysis) and 1,8-diazabicyclo[5.4.0]undec-7-ene (5.1 g, 33.5 mmol) were refluxed in 200 ml hexan-1-ol for 36 h. The resulting dark purple solid was washed with 50 ml acetic anhydride, 10 ml ice-cold acetone and 10 ml pentane, then extracted with chloroform (10 × 200 ml). The resulting green solution was evaporated to yield 320 mg dark green solid, which was purified by HPLC using 1% methanol in dichloromethane as an eluent to yield dark green NdPc 2 (retention time 6.2 min, 13 mg, 11 μmol, 0.3% yield). HPLC was performed on a Waters HPLC system with photodiode array detector equipped with a 250 × 20 mm ProntoSIL 120-10-Si preparative column (10 μm silica particles with a 120-Å pore size). The rate flow of the eluent was 10 ml min −1 . Alternatively, purification could be accomplished by two successive chromatography columns on a silica gel using first 2%, then 1% methanol in dichloromethane as the eluent. The purity of the product was ascertained by infrared [19] , electrospray ionization–mass spectrometry ( m / z =1,168.2 Da, M + ) and ultraviolet–visible ( ε 678 nm =2.10 5 M −1 cm −1 in dichloromethane [27] ). Transmission infrared spectra (KBr pellets) were recorded on a Bruker Vertex 70 spectrometer. Electrospray ionization–mass spectrometry was recorded on the positive mode on a methanol–dichloromethane solution acidified with trifluoroacetic acid using a ThermoFisher Scientific LTQ-Orbitrap XL spectrometer. Ultraviolet–visible absorption spectroscopy was performed on an Analytik Jena Specord S600 spectrometer. Note that the synthesis yields of NdPc 2 were consistently much lower than those for late lanthanide analogues, for example, DyPc 2 , for which we reached the reported values without difficulty. The increased difficulty in obtaining LnPc 2 complexes for early lanthanides was already recognized 25 years ago [19] ; the increasing size of the central ion leads to a decrease of the metal-to-ligand interaction, favouring the formation of the monophthalocyanine complexe PcNd(OAc) 3 (ref. 19 ) and the triple-decker species Ln 2 Pc 3 (ref. 28 ). Experiments The experiments have been carried out in a multichamber ultra-high vacuum system comprising a preparation chamber for substrate cleaning and molecule deposition and an STM operating at 5 K (Omicron LT-STM). STM tips were electrochemically etched from a polycrystalline W wire in NaOH solution and in-situ flashed by electron-beam bombardment for several seconds to remove oxides. The Cu(100) crystal surface was cleaned by several Ar-sputtering and annealing cycles at 1.5 kV and 750 K, respectively. Molecules were evaporated from a Knudsen cell after several days of degassing below the evaporation temperature of 800 K. The evaporation time for single-molecule coverages was 5 s. I ( V ) spectra and d I /d V maps are recorded by modulating the bias voltage (2.7 kHz, 20 mV) and using lock-in detection. d I /d V maps are measured simultaneously with constant current topography images. The bias voltage is applied to the sample, that is, positive bias voltage corresponds to probing unoccupied states. Calculations Spin-polarized, first-principles total-energy calculations have been carried out in the framework of the density functional theory [29] in the Kohn–Sham formulation [30] by using the projector augmented wave method [31] as implemented in the Vienna ab initio simulation package code [32] , [33] . In our study, we used the Perdew–Burke–Ernzerhof [34] exchange-correlation energy functional and the plane-wave basis set includes all plane waves up to a kinetic energy of 550 eV. To account properly for the orbital dependence of the Coulomb and exchange interactions of the Nd 4 f -states, we employed the Perdew–Burke–Ernzerhof+ U method [35] . The Hubbard parameter for the f -states was set to U =2.2 eV to reproduce the experimental d I /d V features, see main text. The NdPc 2 -Cu(100) system was modelled within the supercell approach and contains five atomic Cu layers with the adsorbed molecule on one side of the slab. The ground-state adsorption geometry was obtained by including van der Waals interactions at a semi-empirical level [36] and by relaxing the uppermost two Cu layers and the molecular degrees of freedom until the atomic forces were converged to less 0.001 eV Å −1 . How to cite this article: Fahrendorf, S. et al . Accessing 4 f -states in single-molecule spintronics. Nat. Commun. 4:2425 doi: 10.1038/ncomms3425 (2013).